Fully-printed high-performance organic thin-film transistors and circuitry on one-micron-thick polymer films Thin, ultra-flexible devices that can be manufactured in a process that covers a large area will be essential to realizing low-cost, wearable electronic applications including foldable displays and medical sensors. The printing technology will be instrumental in fabricating these novel electronic devices and circuits; however, attaining fully printed devices on ultra-flexible films in large areas has typically been a challenge. Here we report on fully printed organic thin-film transistor devices and circuits fabricated on 1-μm-thick parylene-C films with high field-effect mobility (1.0 cm 2 V −1 s −1 ) and fast operating speeds (about 1 ms) at low operating voltages. The devices were extremely light (2 g m −2 ) and exhibited excellent mechanical stability. The devices remained operational even under 50% compressive strain without significant changes in their performance. These results represent significant progress in the fabrication of fully printed organic thin-film transistor devices and circuits for use in unobtrusive electronic applications such as wearable sensors. A new class of electronics technology that is extremely lightweight, thin and flexible is attracting attention of researchers worldwide. The evolution from rigid, heavy and thick electronics to new flexible electronics has reached the point whereby ‘imperceptible’ and ‘epidermal’ electronics can be attached to curved and moving surfaces such as the skin of the human body without any concern to the wearer [1] , [2] , [3] . These devices occupy very small volumes and are environmentally friendly. Organic materials possess intrinsic mechanical flexibility due to loose Van der Waals bonds between organic molecules. Flexible devices made from organic materials [4] , [5] have many applications such as in flexible displays [6] , [7] , radio-frequency identification (RFID) tags [8] , solar cells [9] , electronic skin [10] , pressure sensors [11] , [12] , temperature sensors [13] , chemical sensors [14] , [15] , [16] and bio-sensors [14] , [17] . Organic materials have another important advantage: they are soluble in organic solvents and thereby are more suitable for printing processes than inorganic materials [18] , [19] , [20] . Organic electronics that are fully solution processed [21] , [22] , [23] , [24] , [25] , [26] , [27] , [28] , [29] are of great interest because they also enable large area and low-cost electronics. The ability to use these printing processes on very thin (<10 μm) substrates has potential opportunities for unobtrusive electronic applications. Though several novel studies on flexible electronic devices have been reported [1] , [3] , [5] , [7] , [30] , [31] , [32] , none has led to a fully printed fabrication process that can produce devices with good electrical performance characteristics, such as high mobility, high on/off ratio and ideal threshold voltage of near 0 V. Achieving flexible organic electronics based on organic thin-film transistor (TFT) devices fabricated with fully printed processes will be essential for realizing wearable electronic applications that are low in cost and environmentally friendly. In this study, we fabricate organic TFT devices with excellent electrical characteristics and mechanical stability that are fully printed on ultra-flexible polymer films. The fabricated TFT devices and inverter circuits function at operating voltages of 10 V and have relatively high mobility levels (1.0 cm 2 V −1 s −1 ) and high on/off ratios (>10 6 ). Moreover, they exhibit remarkable mechanical stability, whereby the mobility and on/off current levels remain virtually unchanged even under 50% compressive strain. A p-type diode-load inverter is also fabricated, and it exhibits good transfer characteristics. The inverter circuit functions well at low supply voltages, the measured rise/fall times are relatively short (about 1 ms) and can be maintained under 50% compressive strain. Fully printed organic TFTs on ultra-thin substrates New materials developed by Merck were employed for the organic semiconductor, gate dielectric and electrode treatment layers. As already reported by others, these materials provide for good charge transport and stable operation [33] , [34] . As shown in Fig. 1a , the fabricated organic devices are extremely thin and ultra-flexible; their total thickness is less than 2 μm and total weight is only 2 g m −2 . Our devices were fabricated entirely by printing, enabling them to be easily fabricated on a large scale. An example of our printed devices conforming to a human knee ( Fig. 1b ) illustrates their potential in health care and monitoring applications; they can be gently attached to the skin or wrapped around limbs without the wearer perceiving any discomfort. They can be bent or even wrinkled so that they conform to the movements of the human body, which has uneven surfaces and a large range of motion ( Fig. 1b ). The details for each layer of the fabricated devices are shown in Supplementary Fig. 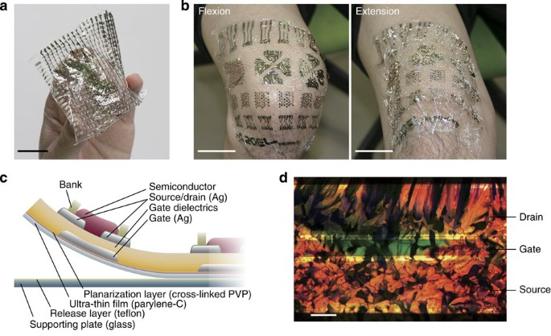Figure 1: Fully printed organic thin-film transistors on ultra-flexible films. (a) A photograph of organic TFT devices on 1-μm-thick parylene-C films. The devices were fabricated entirely with printing processes. Scale bar, 2 cm. (b) Organic device films conforming to a human knee. Scale bar, 4 cm. (c) Cross-sectional diagram of a thin organic TFT device. (d) A polarization microscope image of the channel region. Scale bar, 100 μm. 1 and Supplementary Table 1 . Figure 1: Fully printed organic thin-film transistors on ultra-flexible films. ( a ) A photograph of organic TFT devices on 1-μm-thick parylene-C films. The devices were fabricated entirely with printing processes. Scale bar, 2 cm. ( b ) Organic device films conforming to a human knee. Scale bar, 4 cm. ( c ) Cross-sectional diagram of a thin organic TFT device. ( d ) A polarization microscope image of the channel region. Scale bar, 100 μm. Full size image The parylene-C films are attached to a release layer with weak adhesive strength (13 mN) so that the fabricated devices can be safely peeled off the supporting plates ( Fig. 1c ; Supplementary Fig. 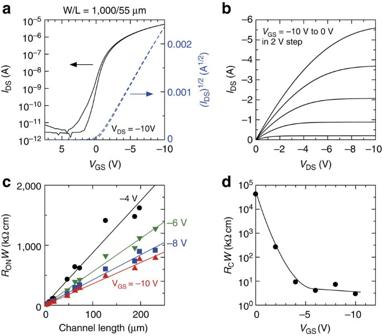Figure 2: Electrical characteristics of fully printed organic TFT devices. (a) Transfer characteristics for fully printed, thin organic TFT device. The plot is of the drain-source current (IDS) as a function of gate-source voltage (VGS) at a drain-source voltage (VDS) of −10 V. The saturation mobility is 1.0 cm2V−1s−1, the on/off ratio exceeds six orders of magnitude. (b) Corresponding output characteristics. The plot is ofIDSas a function ofVDSfor a gate-source voltage from 0 V to −10 V in 2 V steps. (c) Channel width-normalized total on-resistance (RON) as a function of channel length. (d) Width-normalized contact resistance (RC) as a function ofVGS. The width-normalized contact resistance was 3.0 kΩ cm at aVGSof −10 V. 2 and Supplementary Table 2 ). A polarization microscopic image ( Fig. 1d ) shows that the organic semiconductor layers have relatively large crystal domain sizes of ~30 μm, meaning that single-domain crystalline layers can be made to extend across the short channel length region between the source and drain electrodes. These large crystal domains led to the printed organic devices on thin films having excellent electrical characteristics. TFT characteristics Our fabricated devices exhibited excellent ambient air stability, and all of the electrical measurements were performed in ambient conditions. Figure 2a shows the transfer characteristics of a fabricated TFT device, and Figure 2b shows the corresponding output characteristics. The TFT devices exhibited excellent transistor performance at relatively low operating voltages of 10 V. The estimated mobility in the saturation region was 1.0 cm 2 V −1 s −1 , and the on/off ratio exceeded 10 6 . The estimated threshold voltage was –0.53 V, which is near the ideal value of 0 V. We also estimated the contact resistance ( R C ) by using a transfer-line method [35] . For this purpose, we fabricated TFT devices with channel lengths ranging from 5 to 230 μm. The total on-resistance ( R ON ) was taken from the output characteristics. Figure 2c shows width-normalized R ON as a function of channel length. R C was obtained by extrapolating the linear fit to a channel length of zero and plotting it as a function of gate-source voltage ( V GS ) ( Fig. 2d ). R C decreased to as low as 3.0 kΩ cm at V GS =–10 V, a remarkably low contact resistance value for a fully printed organic TFT device and comparable with values for organic TFT devices formed using evaporated metal source/drain electrodes [36] . Such low R C values are attributed to a low energy barrier between the printed organic semiconducting layer and the source/drain electrodes. Figure 2: Electrical characteristics of fully printed organic TFT devices. ( a ) Transfer characteristics for fully printed, thin organic TFT device. The plot is of the drain-source current ( I DS ) as a function of gate-source voltage ( V GS ) at a drain-source voltage ( V DS ) of −10 V. The saturation mobility is 1.0 cm 2 V −1 s −1 , the on/off ratio exceeds six orders of magnitude. ( b ) Corresponding output characteristics. The plot is of I DS as a function of V DS for a gate-source voltage from 0 V to −10 V in 2 V steps. ( c ) Channel width-normalized total on-resistance ( R ON ) as a function of channel length. ( d ) Width-normalized contact resistance ( R C ) as a function of V GS . The width-normalized contact resistance was 3.0 kΩ cm at a V GS of −10 V. Full size image Stability of fully printed TFT devices To demonstrate the robustness of our fully printed organic TFT devices, we conducted several stability tests. 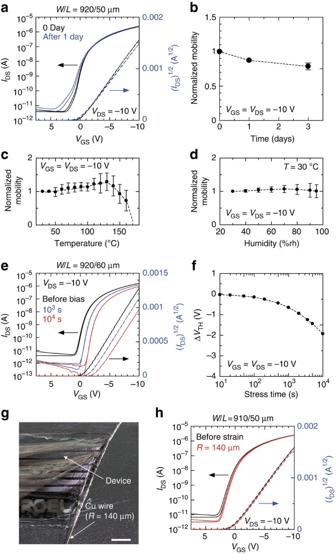Figure 3: Stability of fully printed organic TFT devices. (a) Transfer characteristics of the TFT devices were measured immediately after fabrication (black lines) and after 1 day (blue lines). Even though the TFT devices had no passivation layer, there were only small changes in transistor characteristics. (b) Normalized field-effect mobility as a function of storage time in ambient air conditions. After 3 days, a 21% change in mobility was observed. Error bars in the plots indicate the s.d. (c) Normalized field-effect mobility of the TFT devices as a function of temperature. The mobility on the TFT devices increased up to 130 °C, but began to degrade at >130 °C. Error bars in the plots indicate the s.d. (d) Normalized field-effect mobility of the TFT devices as a function of humidity. The temperature was fixed to 30 °C. Even at high humidity level (95%rh), the transistor devices were functional with almost no observed changes in mobility. Error bars in the plots indicate the s.d. (e) Transfer characteristics of the TFT devices taken before (black line) and after applying a constant bias voltage (VGS=VDS=−10 V) for 103s (blue line) and 104s (red line). (f) Threshold voltage shifts (ΔVTH) as a function of time while applying continuous bias voltages. (g) Photograph of a fully printed organic TFT devices on 1-μm-thick parylene-C films wrapped around a copper wire with a radius of 140 μm. Scale bar, 5 mm. (h) The transfer characteristics of the TFT devices were measured in the bent and unbent states, with no discernible changes in the characteristics due to bending. Figure 3a shows transfer curves of a TFT device immediately after the fabrication process and after 1 day stored in ambient air (about 25 °C, 20% relative humidity). Though slight decreases in on-current and increases of subthreshold swing were observed, the fabricated TFT devices worked very well. Figure 3b shows normalized mobility as a function of storage time. Even after 3 days in ambient air conditions, the changes in mobility amounted to 21%, which verify the relatively long-term air stability of the fully-printed TFT devices. In addition to long-term stability in air, we estimated short-term stability at elevated temperature and moisture levels. The transistor characteristics were measured while the devices were heated by a hot plate. Figure 3c shows the normalized mobility as a function of temperature. The mobility increased slightly at temperatures up to 130 °C, and the TFT device worked well at temperatures as high as 160 °C. We also stored the TFT devices in an environmental test chamber and connected to the semiconductor parameter analyser by external cables, to evaluate their stability in humidity. The temperature in the chamber was fixed at 30 °C, and the humidity levels were changed from 30 to 95%rh and then measured the electrical characteristics. Figure 3d shows normalized mobility as a function of humidity level. Even at high humidity levels (95%rh), the TFT devices clearly worked and almost no changes in mobility were observed. Figure 3: Stability of fully printed organic TFT devices. ( a ) Transfer characteristics of the TFT devices were measured immediately after fabrication (black lines) and after 1 day (blue lines). Even though the TFT devices had no passivation layer, there were only small changes in transistor characteristics. ( b ) Normalized field-effect mobility as a function of storage time in ambient air conditions. After 3 days, a 21% change in mobility was observed. Error bars in the plots indicate the s.d. ( c ) Normalized field-effect mobility of the TFT devices as a function of temperature. The mobility on the TFT devices increased up to 130 °C, but began to degrade at >130 °C. Error bars in the plots indicate the s.d. ( d ) Normalized field-effect mobility of the TFT devices as a function of humidity. The temperature was fixed to 30 °C. Even at high humidity level (95%rh), the transistor devices were functional with almost no observed changes in mobility. Error bars in the plots indicate the s.d. ( e ) Transfer characteristics of the TFT devices taken before (black line) and after applying a constant bias voltage ( V GS = V DS =−10 V) for 10 3 s (blue line) and 10 4 s (red line). ( f ) Threshold voltage shifts (Δ V TH ) as a function of time while applying continuous bias voltages. ( g ) Photograph of a fully printed organic TFT devices on 1-μm-thick parylene-C films wrapped around a copper wire with a radius of 140 μm. Scale bar, 5 mm. ( h ) The transfer characteristics of the TFT devices were measured in the bent and unbent states, with no discernible changes in the characteristics due to bending. Full size image We also evaluated the operational stability of the devices. We estimated the change in threshold voltage (Δ V TH ) as the devices were stressed with constant bias voltages ( V GS = V DS =–10 V) from their transfer characteristics. Figure 3e shows the changes in transfer characteristics before and after stressing the devices for 10 3 and 10 4 s in ambient air. Though the transfer characteristics shifted slightly in the negative direction, the other key electrical parameters such as on/off ratio and field-effect mobility did not change with the negative gate bias stress. Δ V TH as a function of stress time is plotted in Fig. 3f . Δ V TH was 0.65 V after continuously applying voltages for 10 3 s and was 1.9 V after 10 4 s. This level of operational stability is comparable to evaporated (vacuum processed) organic TFT devices [37] . The mechanical bending stability of the devices was also evaluated. Tensile strains were applied to the organic TFT devices. The strains were parallel to the flow of source-drain current, and the electrical performance of the devices was evaluated before and during the application of strain. Figure 3f shows a photograph of a fabricated TFT device tightly wrapped around a copper wire with bending radius of 140 μm. The transfer characteristics were measured in ambient air with and without strain due to bending, as shown in Fig. 3g , such that there was no discernible change in the electrical characteristics during the bending. The change in the on-current was 3.9%, and the change in the mobility was 1.6% with bending and the on/off ratio remained more than 10 5 . The ultra-thin film substrates help reduce the applied strain in the TFT devices, whereby the calculated strain was ~0.5% or less, even when the devices were bent to a radius of 140 μm [38] , [39] . As several research groups have already reported, such a small degree of strain does not significantly change the electrical performance of organic TFT devices [39] , [40] . Large area fabrication of fully printed devices To further demonstrate the advancements we have made, we proceeded to fabricate fully printed devices on ultra-thin flexible substrates over large areas. All organic TFT devices were fabricated into 20 × 20 array on a 10 cm × 10 cm parylene-C film substrate. 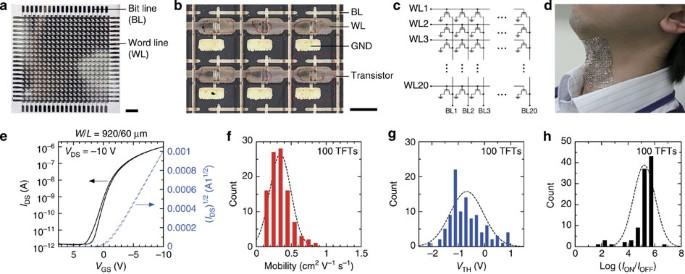Figure 4: Large area TFT array. (a) Top-view photograph of a completed 10 cm × 10 cm fully printed 20 × 20 TFT array fabricated on an ultra-flexible parylene-C film. Scale bar, 1 cm. (b) A magnified view of six TFT devices. Scale bar 2 mm. (c) Circuit diagram of the TFT array. (d) Flexible TFT array sheet conforming to a human throat. (e) Transfer characteristics of a transistor in the array configuration. The saturation mobility is 0.7 cm2V−1s−1atVGS=VDS=−10 V. Although the fabricated TFT array devices had relatively thick dielectric layers (1,500 nm), they operated at low voltages with good mobilities and high on/off ratios. (f–h) Distribution of mobility (f), threshold voltage (g) and logarithmic on/off ratio (h) as-measured results for 100 randomly selected TFT devices in the array. Average mobility was 0.34±0.15 cm2V−1s−1, average threshold voltage was –0.68±0.63 V, and average logarithmic on/off ratio was 5.2±0.8. The dashed lines indicate normal distributions. Figure 4a shows a top-view photograph of the completed 10 cm × 10 cm fully printed array on the parylene-C substrate. A magnified view of six TFT devices is shown in Fig. 4b . The circuit diagram for the fabricated TFT array is shown in Fig. 4c . To prevent shorting of the TFT and to improve device yield, a relatively thick dielectric layer (1,500 nm) was used in the array devices. Here, the average TFT device W/L ratio in the array was 21. An example of a large-area and ultra-flexible device that conforms to the human throat ( Fig. 4d ) illustrates the potential for this technology in sensor in health care and the monitoring of biological parameters. Figure 4e shows transfer characteristics in the array. The transistor exhibited excellent electrical performance with negligible hysteresis. Although a thick dielectric layer was used, the TFT device had sufficiently large on/off ratio (>10 5 ) and relatively high field-effect mobility (0.7 cm 2 V −1 s −1 ) at low operating voltages ( V GS = V DS =–10 V). To analyse this array statistically, 100 TFT devices or 25% of the TFT devices were characterized in terms of electrical performance. The plots in Fig. 4f–h show the distributions of various transistor performance parameters. The mobility in the saturation regime was 0.34±0.15 cm 2 V −1 s −1 on average, and the maximum value was 0.88 cm 2 V −1 s −1 . The average threshold voltage was –0.68±0.63 V and the average logarithmic on/off ratio was 5.2±0.8, which show that the average on/off ratio exceeds a level of 10 5 . These variations in electrical characteristics are comparable to those of obtained with organic TFT devices of same configuration using the same organic semiconducting materials on 125-μm-thick PEN substrates [21] . Figure 4: Large area TFT array. ( a ) Top-view photograph of a completed 10 cm × 10 cm fully printed 20 × 20 TFT array fabricated on an ultra-flexible parylene-C film. Scale bar, 1 cm. ( b ) A magnified view of six TFT devices. Scale bar 2 mm. ( c ) Circuit diagram of the TFT array. ( d ) Flexible TFT array sheet conforming to a human throat. ( e ) Transfer characteristics of a transistor in the array configuration. The saturation mobility is 0.7 cm 2 V −1 s −1 at V GS = V DS =−10 V. Although the fabricated TFT array devices had relatively thick dielectric layers (1,500 nm), they operated at low voltages with good mobilities and high on/off ratios. ( f – h ) Distribution of mobility ( f ), threshold voltage ( g ) and logarithmic on/off ratio ( h ) as-measured results for 100 randomly selected TFT devices in the array. Average mobility was 0.34±0.15 cm 2 V −1 s −1 , average threshold voltage was –0.68±0.63 V, and average logarithmic on/off ratio was 5.2±0.8. The dashed lines indicate normal distributions. Full size image Mechanical robustness of fully printed organic TFT devices The strain stability of the fabricated fully printed organic TFT devices and p-type diode load inverter circuits was evaluated by applying compressive strain. Here, the fabricated devices were released from their supporting plates and laminated on a pre-stretched elastomer (NITOMS, J0930, No.541) by picking them off the plates with tweezers and placing them on the elastomer [1] . When the pre-strained elastomer was relaxed, the adhesion between the elastomer and the thin film caused the strain in the elastomer to transfer to the thin film, forming a network of out-of-plane wrinkles in the device. Details of compression test apparatus are shown in Supplementary Fig. 3 . 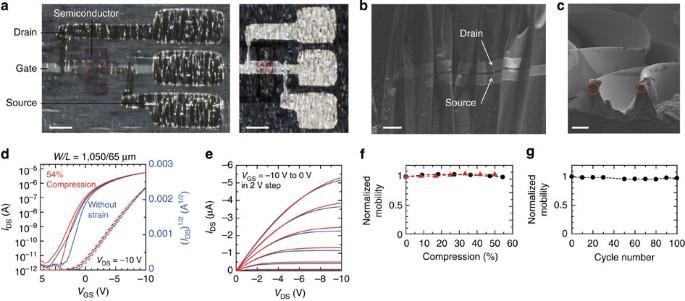Figure 5: Stretch-induced effect of fully printed organic TFT devices. (a) Photos of an ultra-flexible transistors without compression (left) and under 50% compression (right). Scale bars, 1 mm. (b) Top-view SEM image of the fully printed TFT device under 50% compressive strain. Scale bar, 200 μm. (c) Cross-sectional SEM image of a ultra-thin film undergoing 50% compressive strain. The two red circles represent 7 μm (left) and 5 μm (right) bending radii. Scale bar, 20 μm. (d) Transfer characteristics of a TFT device operated under no strain (blue) and 54% compressive strain (red), demonstrating the mechanical stability of the fully printed TFT devices. The mobility decreased slightly from 0.95 to 0.94 cm2V−1s−1under 54% compressive strain, and the threshold voltage shifted from 0.66 to 1.09 V. (e) Corresponding output characteristics. The plot is ofIDSas a function ofVDSfor a gate-source voltage from 0 V to −10 V in 2 V steps. (f) Changes in mobility as a function of compressive strain. The devices were compressed in two directions: perpendicular (black circles) and parallel (red triangles) to the flow ofIDS. The TFT devices showed no degradation under perpendicular and parallel compressive strain. (g) Mechanical durability during repeated compression and relaxation. The normalized mobility was plotted as a function of the number of cycles. Figure 5a shows a picture before and after relaxation of the elastomer. The devices became folded when the elastomer relaxed and the device area was reduced by almost 50% of its initial value. Figure 5b shows surface top-view image of an organic TFT device under 50% compressive strain measured using a scanning electron microscope (SEM). Here, the substrate films were wrinkled and the TFT devices were creased or even folded. Figure 5c shows a cross-sectional SEM image of a transistor under 50% compressive strain. The SEM image reveals that the ultrathin-substrates can be folded to very small bending radii of about 5 μm. We performed the strain experiment in two directions: perpendicular and parallel to the source-drain current flow. Figure 5d shows the transfer characteristics of the TFT device before and after applying compressive strain perpendicular to the flow of I DS . Printed devices typically exhibit problems with mechanical durability because of the lack of adhesive strength on the film surfaces [41] , [42] ; in contrast, these fully printed TFT devices exhibited excellent mechanical stability. There was no apparent degradation in the transfer characteristics. The mobility values were virtually the same (0.95 cm 2 V −1 s −1 without compression, 0.94 cm 2 V −1 s −1 under 54% compression), and the on/off ratio exceeded 10 6 for the device under 54% compression. The threshold voltage shifted slightly in the positive direction, from 0.66 to 1.09 V; this shift is considered to be negligible. The on-current increased from 5.5 to 5.6 μA, which was caused by the shift in threshold voltage. The corresponding output characteristics ( Fig. 5e ) show that the linear characteristics did not change even after the 54% compressive strain, which indicated that there was no change in contact resistance. The plot in Fig. 5f shows the TFT device mobility as a function of compressive strain in directions perpendicular and parallel to the source-drain current flow. No irreversible degradation was observed during these experiments, and the mobility values were virtually unchanged, even after applying a 54% compressive strain. There was no dependence on the direction of strain, which indicates the fabricated transistors had excellent omnidirectional mechanical stability. A stress cycle was also applied to the TFT devices, whereby the devices were repeatedly compressed from 0 to 50% and immediately released to their uncompressed state. This stress cycle was repeated at a rate of three times per minute. The plot in Fig. 5g shows the normalized mobility as a function of the number of compressive strain cycles. Even after 100 full cycles, the TFT device was fully functional and the changes in mobility amounted to <4%. Figure 5: Stretch-induced effect of fully printed organic TFT devices. ( a ) Photos of an ultra-flexible transistors without compression (left) and under 50% compression (right). Scale bars, 1 mm. ( b ) Top-view SEM image of the fully printed TFT device under 50% compressive strain. Scale bar, 200 μm. ( c ) Cross-sectional SEM image of a ultra-thin film undergoing 50% compressive strain. The two red circles represent 7 μm (left) and 5 μm (right) bending radii. Scale bar, 20 μm. ( d ) Transfer characteristics of a TFT device operated under no strain (blue) and 54% compressive strain (red), demonstrating the mechanical stability of the fully printed TFT devices. The mobility decreased slightly from 0.95 to 0.94 cm 2 V −1 s −1 under 54% compressive strain, and the threshold voltage shifted from 0.66 to 1.09 V. ( e ) Corresponding output characteristics. The plot is of I DS as a function of V DS for a gate-source voltage from 0 V to −10 V in 2 V steps. ( f ) Changes in mobility as a function of compressive strain. The devices were compressed in two directions: perpendicular (black circles) and parallel (red triangles) to the flow of I DS . The TFT devices showed no degradation under perpendicular and parallel compressive strain. ( g ) Mechanical durability during repeated compression and relaxation. The normalized mobility was plotted as a function of the number of cycles. Full size image Static and dynamic operation of organic integrated circuits We also evaluated the mechanical stability of unipolar diode-load inverters fabricated on thin parylene-C films. 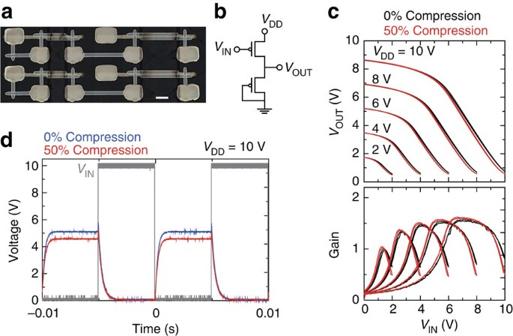Figure 6: Fast operating of printed organic circuits. (a) Photograph of fabricated unipolar organic diode-load inverter circuits. Scale bar, 1 mm. (b) Circuit diagram of the inverter device. (c) Static transfer characteristics of the inverter and small-signal gain as a function of input voltage (VIN). The black solid line indicates the characteristics without strain and the red solid lines indicate those of circuits under 50% compressive strain. (c) Dynamic operation of the inverter circuit. A continuous driving voltage (VDD) of 10 V and an AC input voltage with a 100 Hz rectangular waveform from 0 to 10 V (gray) were applied to the inverter, and the output voltage was monitored using a digital oscilloscope. The blue line indicates the output voltage without strain, and the red line indicates the output voltage under 50% compressive strain. Figure 6a shows a photograph of the inverter circuit, and Figure 6b shows a circuit diagram for the inverter. The ratio between the drive and load transistors is 2.6:1. Both transistors had channel lengths of 20 μm. Figure 6c plots static transfer characteristics measured in ambient air of a diode-load inverter under no compressive strain and under 50% compressive strain. The output voltage ( V OUT ) and small-signal gain were plotted as a function of input voltage ( V IN ). There was no significant change in the electrical characteristics during bending, and the inverter functioned properly even at a driving voltage ( V DD ) of 2 V. The trip point when the inverter was not under compression was 5.92 V at V DD =10 V, and 0.95 V at V DD =2 V, which are close to ideal trip voltages of V DD /2. The small-signal gain of the inverter without compression was 1.57 at V DD =10 V and 0.97 at V DD =2 V. The trip point of the inverter under 50% compressive strain was 5.84 V at V DD =10 V and 0.92 V at V DD =2 V. The small-signal gain of the inverter under 50% compression was 1.61 at V DD =10 V and 1.00 at V DD =2 V. The changes in the trip point and gain in the case of compressive strain were <5% of their values in the case of no compressive strain. Figure 6d shows the dynamic response of the same inverter circuit. We applied a continuous V DD of 10 V and an AC input voltage with 100-Hz rectangular waveform ranging from 0 to 10 V to the inverter and monitored the output voltage using a digital oscilloscope. The measured rise and fall times in the case of no compression were 427 and 691 μs, which corresponds to a total delay time of 1.12 ms. This delay is quite short for fully printed organic circuits, including those fabricated with carbon-nanotube transistors [27] , [28] . The operating speeds remained stable even when compressive strain was applied to the films and the circuits crumpled. The measured rise and fall times of the inverter under 54% compressive strain were 495 and 705 μs, which corresponds to a total delay of 1.20 ms and only a 7% change from the initial total delay. These results exemplify the outstanding mechanical stability of fast-operating printed organic circuits fabricated on thin films. Figure 6: Fast operating of printed organic circuits. ( a ) Photograph of fabricated unipolar organic diode-load inverter circuits. Scale bar, 1 mm. ( b ) Circuit diagram of the inverter device. ( c ) Static transfer characteristics of the inverter and small-signal gain as a function of input voltage ( V IN ). The black solid line indicates the characteristics without strain and the red solid lines indicate those of circuits under 50% compressive strain. ( c ) Dynamic operation of the inverter circuit. A continuous driving voltage ( V DD ) of 10 V and an AC input voltage with a 100 Hz rectangular waveform from 0 to 10 V (gray) were applied to the inverter, and the output voltage was monitored using a digital oscilloscope. The blue line indicates the output voltage without strain, and the red line indicates the output voltage under 50% compressive strain. Full size image Although the fully printed organic TFT devices fabricated on ultra-thin substrates had no passivation layer, the devices exhibited both mechanical robustness and environmental stability. As already reported by several research groups, environmental robustness and stability can be further improved by using the appropriate passivation layer materials to prevent penetration of oxygen or water into the semiconducting layer [43] . These passivation layers also prevent changes in semiconducting layers at high temperatures [44] and embed the semiconducting layer to neutralize strain [4] . The stability of TFT device under temperature and humidity will allow for these devices to attach directly to the human body to monitor biological changes, and their mechanical robustness will allow the devices to attach to highly uneven surfaces with large ranges in motion. Because of their thinness and lightness, our TFT devices can operate even under the influence of wind (see Supplementary Fig. 4 and Supplementary Movie 1 ). Printing processes are sensitive to both surface roughness and wettability of the substrates, requiring control of the substrate surface energy. Although a planarization layer was used in the devices fabricated for this study to improve the substrate surface roughness, the layer could also be used for controlling surface energy of the substrates to a desired level. Therefore, this fabrication technique is compatible with other printing processes, such as gravure printing [45] or screen printing [46] . In conclusion, we have fabricated fully printed organic transistors and inverter circuits on 1-μm-thick polymeric films and have demonstrated their excellent mechanical robustness, environmental stability and potential in large-area flexible devices. The devices are ~1,000 nm thick, so the total thickness of our devices including the substrate is about 2 μm. The devices exhibit excellent stability in air, and at temperature and with humidity. The fabricated devices had excellent static and dynamic electrical characteristics under compressive strains as large as 50%. Further improvements in electrical performance and dynamic responses of these devices will be possible with material developments in the semiconducting and dielectric layers and through the use of more advanced printing technologies. The large-area fabrication of the fully printed TFT devices demonstrated in this study further illustrates the potential to these devices in novel electronic applications, such as large-area sensors. Device fabrication The schematic structure for the organic TFT devices is shown in Fig. 1c . Glass plates (thickness 0.7 mm) were used as supporting carrier plates to ease the handling of the 1-μm-thick Parylene-C films during device fabrication, whereby a solution of fluoropolymer (DuPont, Teflon AF 1600) in Fluorinert (3 M FC-43) was spin-coated onto the glass plates to form a fluoropolymer layer with a thickness of 210 nm. Because of the low surface energy of the fluoropolymer layer (about 8.1 mN m −1 ), the parylene-C layer formed onto the fluoropolymer layer can be readily peeled from the supporting glass plates without causing damage. The 1-μm-thick parylene-C (KISCO, diX-C) films were formed by chemical vapour deposition. Dichloro-p-xylylene powders were sublimed at 135 °C in a sublimation chamber and were converted into monomer gas at 650 °C in a pyrolysis chamber. The monomers were deposited onto the plates and polymerized to form polymer films of poly-p-xylylene in a deposition chamber with a base pressure of <35 mTorr. These ultra-thin films had a surface roughness of about 4 nm (rms) (see Supplementary Fig. 1 and Supplementary Table 1 ). A crosslinked poly(4-vinyl-phenol) (PVP) material was used as a planarization layer for the films. PVP (Mw~25,000, Sigma Aldrich) and poly(melamine-co-formaldehyde) (Mn~432, 84 wt%, Sigma Aldrich) as a crosslinking agent were mixed in propylene glycol monomethyl ether acetate (PGMEA). The parylene-C films were coated with an 130 nm crosslinked PVP layer to reduce surface roughness, which was deposited by spin-coating and cured at a temperature of 150 °C. The surface roughness of the planarization layer was 0.18 nm (rms). The surface of the crosslinked PVP layer was then treated for 1 min in oxygen plasma to alter the surface wettability (plasma power was 100 W). The surface roughness after the treatment was 0.23 nm (rms), which is sufficient smoothness for fabricating organic TFT devices on the films. Next, silver (Ag) nanoparticle ink in an aqueous solvent (DIC Japan, JAGLT-01) was patterned into the gate electrodes on the film by using an inkjet printer (Fujifilm Dimatix, model DMP2831) with a print head having 10 pl nozzles. The Ag nanoparticle ink was printed using a customized waveform, and the droplets were deposited with a dot-to-dot spacing of 60 μm. During the inkjet patterning process, the substrate temperature was maintained at 30 °C. After printing, the substrates were stored for 30 min in an environmental test chamber (ESPEC, model SH-221), within which the temperature was maintained at 30 °C, and relative humidity was kept at 95%rh to planarize the electrodes [47] . After the drying process, the substrates were heated at 120 °C for 1 h to sinter the silver nanoparticles. The fabricated silver gate electrodes had a uniform thickness of about 100 nm. After forming these electrodes, a solution of polymer dielectric materials (Merck, lisicon D207) was spin-coated to form gate dielectric layers. After spin coating of the dielectric layer, the substrates were heated at 120 °C for 1 min on a hotplate and then crosslinked by using a UV treatment (USHIO, model UX-3). The wavelength of UV radiation was 365 nm, and the dosage was 2,650 mJ cm −2 . The thickness of dielectric layers for individual TFT devices and circuits was 360 nm and 1,500 nm for the large area TFT array devices with thicker dielectric layers. Silver nanoparticle ink in a tetradecane-based solvent (Harima Chemicals, NPS-JL) was patterned with an inkjet printer to form the source/drain electrodes. The droplets were deposited with a dot-to-dot spacing of 60 μm. The TFT device geometry was defined by the patterning data for the inkjet printing process. After that, a self-assembled monolayer (SAM) treatment for source/drain electrodes (Merck, lisicon M001) was prepared by dipping the substrate into a solution of propanol for 1 min. The SAM treatment changed the work function of the printed silver source/drain electrodes from 4.7 to 5.3 eV, which reduces the energy barrier between the organic semiconducting layer and the source/drain electrodes [48] . The SAM modification process results in significant improvements to the transistor performance [21] . Next, a solution of fluoropolymer (DuPont, Teflon AF 1600) in Fluorinert (3 M, FC-43) was used as a bank layer and was patterned using dispenser equipment (MUSASHI Engineering, Image Master 350 PC), which includes a three-axis table and an air dispenser, both of which are computer-controlled to precisely dispense and pattern the solution. The 200-nm-thick fluoropolymer bank layers were printed at a patterning speed of 20 mm s −1 and with a discharge pressure of 5 kPa. During the dispenser patterning process, the platen and nozzle temperatures were maintained at 30 °C. After printing the bank layer, the substrates were stored in an air ambient for 10 min to remove the solvent. The final step in the process was formation of the organic semiconducting layer; a mesitylene-based formulation of a soluble small-molecule p-type organic semiconducting material (Merck lisicon S1200) with a deep ionization potential of 5.4 eV (refs 21 , 33 , 34 ) was printed onto the area defined by the bank layer by using dispenser equipment at a patterning speed of 20 mm s −1 and discharge pressure of 1 kPa. During the dispenser patterning process, the platen and nozzle temperatures were maintained at 30 °C. After patterning the semiconducting layer, the substrates were baked at 100 °C for 1 min on a hotplate. Device characterization The electrical characteristics of the fabricated capacitors and TFT devices were measured by using a semiconductor parameter analyser (Keithley, model 4200-SCS). All electrical measurements on the organic TFT devices were carried out in air ambient. The surfaces of the fabricated devices were observed using a laser microscope (Olympus, model OLS-4000) and polarization microscope (Nikon ECLIPSE ME600). The work function of the source/drain electrodes was measured using photoemission spectroscopy (Riken Keiki, model AC-3). The adhesion strength of the parylene-C films was measured using a scratch method (RHESCA, CSR-2000). How to cite this article: Fukuda, K. et al. Fully-printed high-performance organic thin-film transistors and circuitry on one-micron-thick polymer films. Nat. Commun. 5:4147 doi: 10.1038/ncomms5147 (2014).